Angular momentum-induced circular dichroism in non-chiral nanostructures Circular dichroism, that is, the differential absorption of a system to left and right circularly polarized light, is one of the only techniques capable of providing morphological information of certain samples. In biology, for instance, circular dichroism spectroscopy is widely used to study the structure of proteins. More recently, it has also been used to characterize metamaterials and plasmonic structures. Typically, circular dichorism can only be observed in chiral objects. Here we present experimental results showing that a non-chiral sample such as a subwavelength circular nanoaperture can produce giant circular dichroism when a vortex beam is used to excite it. These measurements can be understood by studying the symmetries of the sample and the total angular momentum that vortex beams carry. Our results show that circular dichroism can provide a wealth of information about the sample when combined with the control of the total angular momentum of the input field. Since its discovery in the nineteenthth century, circular dichroism (CD) has been widely used in science. Defined as the differential absorption of left and right circular polarization (LCP or RCP) [1] , its uses are as diverse as protein spectroscopy, DNA studies and characterization of the electronic structure of samples [2] . In some cases, when the CD signal is too weak, a variation of CD is used in exciting the sample with a strong magnetic field oriented parallel to the direction of light propagation [3] , [4] . This variation, known as magnetic CD, can detect some transitions and paramagnetic phenomena that are too weak to be seen with conventional CD. In the advent of nanophotonic circuitry, a lot of work has been put recently into characterizing plasmonic components in terms of both techniques, but especially CD [5] , [6] , [7] , [8] . Typically, it was thought that samples that produced CD had to be chiral, that is, they could not be superimposed with its mirror image [9] . However, recent experiments with planar mirror-symmetric plasmonic structures have shown that a non-zero CD can be obtained if the sample is illuminated at oblique angles [10] , [11] , [12] , [13] . Other attempts to create CD with a non-chiral sample have been carried out surrounding the sample with a chiral medium [14] , [15] , [16] . In this article, we show for the first time how to induce CD in a non-chiral sample, under normal incidence. In contrast to the previous approaches, the mirror symmetry of the system is broken with an internal degree of freedom of the input beam: its angular momentum (AM). The AM of light has gained a lot of interest since the seminal work of Allen et al . [17] One of the interesting properties of the AM of light is that photons carry AM in packets of m ℏ units. Furthermore, it was shown that the AM of a beam is linearly related to the rotation speed that absorbing particles can achieve when they interact with the beam [18] . Our experiments show that CD can be induced in a non-chiral sample if the two (left and right) circularly polarized modes are vortex beams. The reason behind this interesting phenomenon is that the input beams are not mirror images of each other. Experimental set-up A sketch of the experimental set-up we used is depicted in Fig. 1 . It can be divided into three parts: preparation of states, non-paraxial interaction with the sample and measurement. For the state preparation we use a CW laser working at wavelength λ 0 =633 nm, producing a collimated, linearly polarized Gaussian beam. From this Gaussian beam, we create a vortex beam (see Fig. 1c ) with a spatial light modulator (SLM) by displaying an optimized pitchfork hologram [19] (see Fig. 1b ). Proper control of the pitchfork hologram allows us to create a phase singularity of order q in the centre of the beam, that is, the phase of the beam twists around its centre from 0 to 2 πq radians in one revolution. Note that when q =0, the SLM behaves simply as a mirror. We finish the preparation of the input beam by setting its polarization to either LCP or RCP. This change of polarization does not appreciably affect the spatial shape of the input beam. 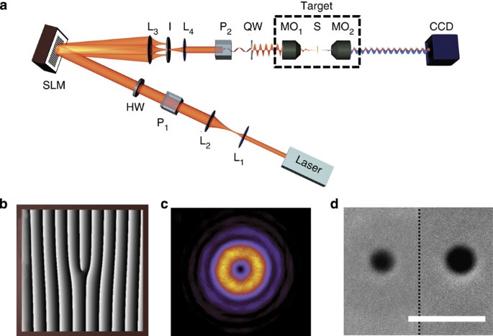Figure 1: Schematic view of the optical set-up in consideration. (a) Both a left and a right circularly polarized vortex beam goes through a subwavelength circular aperture and their transmissivities are measured. First, we prepare an input Gaussian beam from a laser source in order to optimize the diffraction from the SLM. We expand it to match the size of the SLM chip with a telescope (lenses L1–L2) and then we control its polarization with a polarizer (P1) and a half wave plate (HW). A pitchfork-like hologram (b) is used to prepare a vortex beam (c) and the non-desired orders of diffraction are filtered with a lens (L3) and an iris (I). Lens L4is used to match the size of the back aperture of the microscope objective. Then, we control its circular polarization with a second polarizer P2and a quarter wave plate QW. After that, we focus the beam to the plasmonic structure (S) (d) with a microscope objective (MO1) of NA=1.1. The scale bar indis 1-μm long. Finally, we collimate the scattered light from the sample with another microscope objective (MO2) with NA=0.9 and measure the transmission with a charged-couple device (CCD) camera. Figure 1: Schematic view of the optical set-up in consideration. ( a ) Both a left and a right circularly polarized vortex beam goes through a subwavelength circular aperture and their transmissivities are measured. First, we prepare an input Gaussian beam from a laser source in order to optimize the diffraction from the SLM. We expand it to match the size of the SLM chip with a telescope (lenses L 1 –L 2 ) and then we control its polarization with a polarizer (P 1 ) and a half wave plate (HW). A pitchfork-like hologram ( b ) is used to prepare a vortex beam ( c ) and the non-desired orders of diffraction are filtered with a lens (L 3 ) and an iris (I). Lens L 4 is used to match the size of the back aperture of the microscope objective. Then, we control its circular polarization with a second polarizer P 2 and a quarter wave plate QW. After that, we focus the beam to the plasmonic structure (S) ( d ) with a microscope objective (MO 1 ) of NA=1.1. The scale bar in d is 1-μm long. Finally, we collimate the scattered light from the sample with another microscope objective (MO 2 ) with NA=0.9 and measure the transmission with a charged-couple device (CCD) camera. Full size image After this initial preparation, the light is focused down to interact with a plasmonic sample using a high numerical aperture (NA=1.1) microscope objective. The samples are circular nano-apertures drilled in a 200-nm gold film deposited on a 1-mm glass substrate (see Fig. 1d ). The diameters of the nano-apertures range from 200 to 450 nm (see Methods). They are centred with respect to the incident beam with a nano-positioning stage. The interaction of the light and the centred nano-aperture occurs in the non-paraxial regime. Typically, the nano-aperture only allows a small part of the incoming beam to be transmitted. The transmitted light is scattered in all directions. This facilitates the coupling of light to superficial modes of light, as it has been described theoretically and experimentally by many authors [20] , [21] , [22] . The transmitted light is then collected by another microscope objective. Finally, a camera is used to capture the transmitted intensity. The CD of our samples is measured using the following procedure: first, we create a vortex beam of optical charge q with the SLM. Second, we rotate QW to polarize the beam with LCP. Then, we centre the sample with respect to the beam, at the focal plane of MO 1 . We measure the transmitted intensity , where L stands for the polarization of the beam (LCP) and q for its optical charge. Then, we rotate QW again to change the polarization state to RCP and re-centre the sample. At last, we measure the transmitted intensity . From there, the CD associated to the vortex beam with charge q can be obtained in the usual manner: the transmitted intensity with LCP and RCP modes are subtracted and the result is normalized by their addition: Experimental results Our results are presented in Table 1 and Fig. 2 . The first column of Table 1 shows the size of the nano-aperture under consideration. The rest of the columns show the measured CD using beams with different phase singularities of order q =−1, 0, 1, respectively. As expected, because of the fact that the circular nano-aperture is mirror-symmetric and the incidence is normal, the CD is very close to zero when the incident beam is Gaussian ( q =0). The residual CD can be attributed to small asymmetries on the sample or the incoming beam. When vortex beams with q =−1, 1 are used, the situation is very different. We obtain a very large value for the CD, of the order of 90% for some nano-apertures, even though the incidence is normal and the nano-aperture is still mirror-symmetric. Furthermore, it can be observed that there is an underlying symmetry relating the value of CD 1 and CD −1 . Indeed, CD 1 ≃ CD −1 . Table 1 Measurements of circular dichroism CD (%) for three different phase singularities q as a function of the diameter of the nano-aperture. 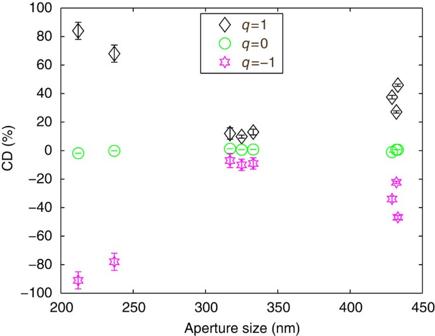Figure 2: Measurements of CD (%) for three different phase singularitiesqas a function of the diameter of the nano-aperture. CD is computed using equation (1). Black diamonds are used to represent the CD obtained withq=1; green circles forq=0 and magenta hexagon stars forq=−1. Error bars are computed as the standard deviation of a set of 20 measurements with the same sample. The most probable source of this error are vibrations of the mechanical system, which misalign the sample with respect to the incident beam. In contrast, the larger differences between samples of roughly the same size are probably due to discrepancies in their geometry (eccentricity and ellipticity). Full size table Figure 2: Measurements of CD (%) for three different phase singularities q as a function of the diameter of the nano-aperture. CD is computed using equation (1). Black diamonds are used to represent the CD obtained with q =1; green circles for q =0 and magenta hexagon stars for q =−1. Error bars are computed as the standard deviation of a set of 20 measurements with the same sample. The most probable source of this error are vibrations of the mechanical system, which misalign the sample with respect to the incident beam. In contrast, the larger differences between samples of roughly the same size are probably due to discrepancies in their geometry (eccentricity and ellipticity). Full size image Let us now discuss the results presented in Table 1 and Fig. 2 . In order to understand the appearance of CD in a circular sample under normal incidence, we have to take a careful look at the symmetries of the system and the light probing the samples. We can start considering the symmetries of the target T comprising the two microscope objectives MO 1 , MO 2 and the sample S (see Fig. 1a ). This will simplify the discussion, as we will just consider the interaction of a paraxial beam with T , as well as the output beams that will also be paraxial. Then, as both the circular nano-aperture and the microscope objectives have cylindrical symmetry along an axis normal to them, T is cylindrically symmetric. Without loss of generality we will label the symmetry axis as z and we will denote the rotations around this axis by R z . Furthermore, T is also symmetric under any mirror transformation that contains the z axis, for example, a transformation flipping the x axis and leaving the other axes invariant. We will refer to such transformations as . Now we will turn our attention to the symmetries of the light beams. The electric field of the light beam incident on T can be described within the paraxial approximation with the complex vector: where , and being the horizontal and vertical polarization vectors, respectively, A is a normalization constant, | k 0 |=2 π/λ 0 with λ 0 the wavelength in consideration and ρ , φ , z are the cylindrical coordinates. An implicit harmonic exp(− i 2 πct / λ 0 ) dependence is assumed, where c is the speed of light. Note that p =1 refers to LCP and p =−1 to RCP. Now, if we apply a rotation around the z axis by an angle θ to this beam, the resulting beam acquires a constant phase: . These kinds of beams are then eigenstates of the generator of rotations around the z axis, that is, the z component of the total AM J z : . The J z eigenvalue is m = p + q . In addition, note that a beam with p =0 would be linearly polarized and will be no longer an eigenstate of J z , since a rotation of the field would not leave it invariant. Within the paraxial approximation, the beams with p =±1 are also eigenstates of the helicity operator Λ (refs 23 , 24 , 25 ). That is, , where Λ= J · P /| P | and P is the linear momentum operator. Hence, with our notation, a beam with p =1 is both LCP and also an eigenvector of Λ with value 1, whereas a beam with p =−1 is RCP and its helicity equals to −1. We would like to emphasize that this simple relation between helicity and polarization is only valid because, as mentioned previously, we are describing the system in the paraxial regime [26] . When the paraxial approximation does not hold, the polarization of the field and helicity can no longer be so simply related [24] . Now, if we apply a mirror transformation to the incident beam we obtain: where α is a phase given by the specific mirror transformation chosen. That is, we obtain a beam with the AM and the helicity eigenvalues flipped. This is a consequence of the fact that both J z and Λ anticommute with the mirror symmetry transformations (ref. 27 ): and . We will now explain our experimental results. We will start by classifying the transmitted electric field with the parameters p and q from the incident field: p =−1, 1 and q =−1, 0, 1. Remember that for the incident field , p is modified with QW and q with the SLM (see Fig. 1 ). Mathematically, the field can be obtained through the use of a linear operator, , which can be found using the Green dyadic formalism and contains all the relevant information about target T (refs 21 , 28 ). That is, , where the action of on the incident field will in general be in the form of a convolution. As is simply the mathematical description of T , inherits the symmetries of T . Thus, because of the cylindrical and mirror symmetries of the target and given an incident field , the following statements hold: first, the transmitted field will also be an eigenstate of J z with the same eigenvalue of m = p + q (see Methods). Second, two incident beams that are mirror images of each other will produce two transmitted fields that will be mirror images (see Methods). That is, given two mirror-symmetric beams such as and (see equation (3)), their transmitted beams and will be connected via a mirror symmetry: . The proof can be found in Methods, but the physical idea is the following one: the invariance of the system under mirror transformations links the output of mirror-inverted inputs. This last result is the key point to understand our CD measurements with vortex beams presented in Table 1 and Fig. 2 . In equation (1), the intensities can be obtained from the transmitted electric field: where the integral is taken on the plane of the detector (in our case CCD chip of the camera). Then, for a mirror-symmetric sample, it can be proven (see Methods) that Let us apply it to prove that CD 0 =0 and that CD q =− CD − q . When q =0, we obtain that . Substituting this in the definition of CD, equation (1) gives us CD 0 =0. However, when q ≠0, equation (5) leads us to , which implies that CD q =−CD − q , in very good agreement with our measurements. Powerful as these symmetry considerations are, they still cannot explain the quantitative results of CD we obtained, nor their variation with the diameter of the nano-aperture. Note that, in our experiments, the vortex-induced CD 1 varies greatly for different aperture sizes. Thus, holes ~220 nm have a CD close to 90%, while those with sizes ~320 nm present a much lower CD ~10%. Interestingly, the trend is not monotonous and CD 1 increases again to 22% for nano-apertures of 430 nm. The symmetry arguments only indicate that when q ≠0 the two opposite circular polarizations are not the mirror images of each other and then the associated CD q does not have to be zero. Here the AM of light plays a crucial role again. In general, it can be observed that CD measurements compare the differential ratio of electromagnetic fields with opposite circular polarization and a difference of AM of 2 units. For example, CD q =1 relates and , whose respective AM values are m p =1 =1+1=2 and m p =−1 =1−1=0. It is then interesting to observe that CD can also be sensitive to differential absorption of AM states. In the case of the nano-aperture, this is the most probable cause of the giant value of CD obtained in the experiments. Even though the sample is cylindrically symmetric, thus preserving the AM of field, input beams with different values of AM have very different scattering amplitudes. This is very similar to what happens in the scattering from spherical objects, where different spherical modes (the so-called multipolar modes) are scattered with different amplitudes (the Mie coefficients). This problem can be analytically studied using the Generalized Lorenz-Mie Theory [29] , [30] . Using the model of the aplanatic lens [31] , [32] one can check that the fields at the focal plane of MO 1 produced by and are very different (see Fig. 3b ). Consequently, their multipolar decompositions [33] , [34] are different as well. These two dissimilar focused fields couple very differently to the multipolar moments of the structure. In the case of a spherical object, the coupling of multipolar modes depends drastically on its diameter. Furthermore, the relation between the coupling coefficient and the sphere radius is non-linear and rather complex [34] , giving rise to the so-called Mie resonances in the scattering of the sphere. Then, given two spheres of different sizes, different coupling scenarios can occur not only depending on the geometry of the particles but also on the beams used to excite these particles. In fact, similar effects have been experimentally observed for other plasmonic structures [35] , [36] , [37] . 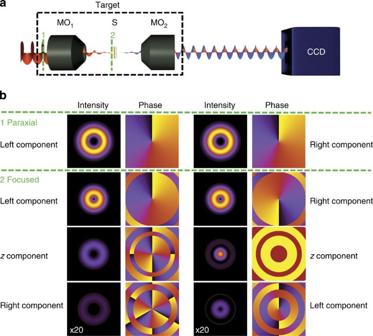Figure 3: Intensity, polarization and phase of a paraxial versus focused beam. (a) Measurement part of the set-up. A paraxial beamis focused by MOon the sample. Then, MOcollimates the transmitted light andis measured with a CCD camera. (b) Intensity and phase plots of the two beams used to carry out the measurement of CDq=1, that is,and. In the upper row, the intensity and phase of the beams are shown on the back aperture plane of the MO1. Both the intensity and the phase can be described with equation 2. In contrast, the three rows below show the intensity and the phase of the same beams (and) at the focal plane of MO1. As it can be observed, even though their paraxial intensities and phases are analogous, their structure is completely different at the focal plane. This is a direct consequence of the fact that the AM of both beams differ in two units. Figure 3: Intensity, polarization and phase of a paraxial versus focused beam. ( a ) Measurement part of the set-up. A paraxial beam is focused by MO on the sample. Then, MO collimates the transmitted light and is measured with a CCD camera. ( b ) Intensity and phase plots of the two beams used to carry out the measurement of CD q =1 , that is, and . In the upper row, the intensity and phase of the beams are shown on the back aperture plane of the MO 1 . Both the intensity and the phase can be described with equation 2. In contrast, the three rows below show the intensity and the phase of the same beams ( and ) at the focal plane of MO 1 . As it can be observed, even though their paraxial intensities and phases are analogous, their structure is completely different at the focal plane. This is a direct consequence of the fact that the AM of both beams differ in two units. Full size image Now, the fact that CD 1 increases from 10 to 25% clearly indicates that the nano-apertures are in this multipolar regime [34] , [38] . If the experiment was conducted with larger apertures (non-subwavelength), the result of the CD measurement would monotonously tend towards 0. Indeed, as the size of the scatterer is increased with respect to the wavelength, the problem can be described with diffraction theory, where the polarization of light does not play any role. In addition, the beams would have to be less focused to interact with the aperture, otherwise they would just go through it. That would make their intensity and phase profiles much more alike, as shown in Fig. 3b . Last but not the least, notice that the sign of CD is positive for q =1, and negative for q =−1. That is, it appears that the transmission of modes with | J z |=2 is larger than the transmission of modes with | J z |=0, regardless of their helicity content. Now, looking at the intensity distribution of these modes at the focal plane, this result seems counter-intuitive. Figure 3b shows the intensity distribution of a mode with | J z |=2 (left) and a mode with | J z |=0 (right). One could argue that the mode with | J z |=2 should transmit more intensity through the nano-aperture as the intensity of its z component is non-null in the centre. Certainly, this effect has been largely studied in STED microscopy. It is known that a non-null z intensity component in the centre has a detrimental effect for the resolution of the technique [39] , [40] . Nevertheless, when using core–shell nanoparticles to enhance the resolution of STED the same conclusion cannot be drawn [41] , [42] . More importantly, Kindler et al . [43] showed that radial and azimuthally polarized beams have different transmissions through a nanohole. In particular, in this work it is shown that an azimuthally polarized beam (which has null intensity in the centre) can have a higher transmission than the radially polarized beam (which has a strong z component with a non-null intensity in the centre) for nanoholes in the range that we probed. In conclusion, we have observed a giant CD on a subwavelength circular aperture induced by vortex beams. We studied the transmission of beams with three different phase singularities of order q =−1, 0, 1. Higher | q | have not been used as the cylindrical symmetry of the beam is experimentally broken when they are focused [44] , [45] . We have seen that the results can be elucidated from a symmetry perspective. In particular, we have proved that, even for mirror-symmetric systems, CD can be induced if the LCP and RCP beams are not connected via a mirror symmetry. Similar results could have been obtained for our samples had we measured an ‘orbital’ dichroism, defined as , that is inverting the azimuthal phase of the paraxial mode, instead of its polarization. Indeed, using equation (5), it can be proven that and for mirror-symmetric samples. This fact reinforces the point that CD measurements are sensitive to the differential absorption of AM states. That is, we show that the information carried by CD measurements has two different contributions: the differential scattering of different circular polarization states but also the differential scattering of different AM states. Notice that equation (5) and the relations between and CD q above will no longer be valid if the sample in use is chiral. A chiral sample interacts differently with the two orthogonal circular polarizations; therefore, the absorption of and will yield different results. A work along these lines was presented by Löffler et al . [46] Thus, we expect that vortex beam-induced CD will be able to unveil properties of non-chiral samples that are hidden to the standard CD measurements. Finally, it is interesting to see that in other related phenomena, such as molecular optical activity, the interplay between the two symmetries associated to helicity and AM (electromagnetic duality and rotational symmetry) are also essential to fully understand the problem from first principles [47] . Preservation of J Z for the transmitted field We consider the rotation transformations ( R z ), mirror transformations ( ) and AM ( J z ) operators, as well as the scattering operator ( ) as linear integrodifferential operators acting on the electric vector of the complex electromagnetic field. Owing to the invariance of T under rotations around the z axis, the linear operator , which contains all the information about the system, commutes with the rotations R z : . Owing to the bijective properties of the exponential function, the same commutation relation holds for the generator of rotations, J z : . Then, given that is an eigenvector of J z , must also be an eigenvector of J z with the same eigenvalue: Scattering of mirror-symmetric beams Owing to the invariance of T under mirror symmetries, the linear operator , which contains all the information about the system, commutes with : . Now, given two mirror-symmetric beams such as and (see equation (3)), it can be checked that their respective transmitted fields ( and ) are related with a mirror symmetry: Proof of As mentioned in the body of the manuscript, the target is cylindrically symmetric scatterer. Hence, if the incident field is an eigenstate of J z with eigenvalue ( p + q ), then the transmitted field needs to remain an eigenstate of J z with the same eigenvalue ( p + q ). Nevertheless, the helicity is, in general, not preserved in the interaction. This phenomenon is a consequence of the duality symmetry being highly broken by the nano-aperture and the multilayer system [24] , [25] , [48] , [49] . Because duality symmetry is highly broken by the sample, the helicity of the incident beam is not preserved. Thus, the field comprises two helicity components, one of polarization and another one of polarization : where and are the complex amplitudes of the two polarizations at the plane of the camera. We call the direct component, as it maintains the polarization state . The other orthogonal component is , and we call it crossed component. The crossed component has a polarization state when the incident state is . Now, we can use the definition of on equation (4), the decomposition of in its two orthogonal components given by equation (8), and the fact that to obtain that can be expressed as: Following an identical procedure, the following equation yields for : Choosing the mirror-symmetric operator to be , we can use equation (3) to get a relation between the coefficients in equations (9 and 10): which implies that and because of the orthogonality of and . Consequently, it follows that: as the integrations limits remain the same under the change . Fabrication of samples The tested nanoholes were fabricated by milling with a focused ion beam (FIB) on a gold layer of 200 nm, deposited on top of a 1-mm-thick glass substrate. The distance between them is 50 μm, thus avoiding the coupling of surface plasmons launched from one nanohole to the closest neighbour. Imaging of the samples The images were taken with a secondary electron scanning electron microscope (JEOL JSM-6480) operated at 10 keV. The images were analysed with Matlab where the boundaries of the nanoholes were determined by selecting the pixels whose intensity was below the 10% of the maximum. The presented images on Fig. 1 were not post-processed. The obtained diameters are listed in Table 1 on the manuscript. Nano-positioning system The sample is mounted on a piezo electric transducer on closed-loop with resolution below 0.5 nm (translation range 300 μm with 20-bit USB interface and noise floor of tens of picometers). How to cite this article: Zambrana-Puyalto, X. et al . Angular momentum-induced circular dichroism in non-chiral nanostructures. Nat. Commun. 5:4922 doi: 10.1038/ncomms5922 (2014).